Chromatin retention of DNA damage sensors DDB2 and XPC through loss of p97 segregase causes genotoxicity DNA damage recognition subunits such as DDB2 and XPC protect the human skin from ultraviolet (UV) light-induced genome instability and cancer, as demonstrated by the devastating inherited syndrome xeroderma pigmentosum. Here we show that the beneficial DNA repair response triggered by these two genome caretakers critically depends on a dynamic spatiotemporal regulation of their homeostasis. The prolonged retention of DDB2 and XPC in chromatin, because of a failure to readily remove both recognition subunits by the ubiquitin-dependent p97/VCP/Cdc48 segregase complex, leads to impaired DNA excision repair of UV lesions. Surprisingly, the ensuing chromosomal aberrations in p97-deficient cells are alleviated by a concomitant downregulation of DDB2 or XPC. Also, genome instability resulting from an excess of DDB2 persisting in UV-irradiated cells is prevented by concurrent p97 overexpression. Our findings demonstrate that DNA damage sensors and repair initiators acquire unexpected genotoxic properties if not controlled by timely extraction from chromatin. Exposure to the ultraviolet (UV) radiation of sunlight induces DNA lesions such as cyclobutane pyrimidine dimers (CPDs) and (6-4) pyrimidine–pyrimidone photoproducts (6-4PPs), which, if not repaired, lead to sun hypersensitivity, genome instability and skin cancer [1] , [2] , [3] , [4] . Excision of this highly mutagenic DNA injury occurs by the nucleotide excision repair (NER) pathway, which depending on the precise lesion location is triggered by two distinct DNA damage recognition routes. The transcription-coupled NER reaction is initiated by RNA polymerase II (POLII)-blocking lesions and, therefore, removes DNA damage exclusively from the transcribed strand of active genes [5] , [6] . In contrast, the global-genome NER reaction takes advantage of the lesion sensors DDB2 (for damaged DNA-binding 2) and XPC (for xeroderma pigmentosum group C) to recognize and remove DNA damage from both transcribed and non-transcribed templates across the whole genome [7] , [8] . Although XPC is the core sensor that detects a wide range of helix-distorting photoproducts and DNA adducts independently of the exact nature of the offending damage [7] , [9] , [10] , DDB2 is an accessory NER subunit that specializes on the recognition of UV-induced CPDs and 6-4PPs [11] , [12] , [13] , [14] , [15] . In addition to interacting with XPC [16] , [17] , DDB2 associates with DDB1 thereby forming a heterodimer, designated as UV-DDB, that provides a bridge for the recruitment of cullin 4A/B (Cul4A/B)-RING ubiquitin ligases [16] , [18] , [19] , [20] , [21] , [22] . Following UV radiation, the major source of genome instability in human skin, the UV-DDB and Cul4A/B ubiquitin ligase complexes move to DNA lesions and ubiquitinate various acceptor proteins including DDB2 and XPC. However, the role of this ubiquitination reaction and its link to the cellular DNA damage response remained elusive and, in particular, it was enigmatic why, by this process, UV radiation induces the degradation of most DDB2 subunits well before excision of the arising photoproducts is completed [23] , [24] . The ubiquitin-selective p97 segregase, also known as valosin-containing protein (VCP) or Cdc48 in yeast, is an ATP-driven molecular chaperone that drives the remodelling of ubiquitinated proteins to facilitate their degradation or recycling [25] , [26] . Chromatin-associated functions of p97 include extraction of the Aurora B kinase from mitotic chromosomes [27] or release of the alpha2 and L3MBTL1 repressors from DNA targets [28] , [29] . Previous reports that the p97 segregase is involved in the remodelling of transcription [30] or replication machineries stalling at UV lesions [31] , [32] , [33] , [34] , [35] , [36] , prompted us to test whether DDB2 and XPC, once ubiquitinated after UV irradiation, may become susceptible to regulation by this multifunctional chaperone. We found that the p97 segregase recognizes ubiquitinated DDB2 and XPC, and that its recruitment to UV lesions, in addition to Cul4A ubiquitin ligase activity, requires the ubiquitin-binding adaptors Npl4, Ufd1 and UBXD7. Failure to remove ubiquitinated DDB2 or XPC, upon p97 depletion or expression of a segregase-inactive p97 mutant, causes retention of both DNA damage sensors in chromatin and impairs the NER reaction, thereby leading to chromosomal aberrations after exposure to UV light. This report thus reveals that the early DNA damage sensors DDB2 and XPC function as a double-edged sword, as they are essential to trigger a beneficial DNA repair activity but, if allowed to accumulate in damaged chromatin without control by the p97 segregase, may become detrimental to the genome. Ubiquitin-dependent recruitment of p97 to UV lesions To monitor the recruitment of p97 complexes to UV lesions, spots of local damage were generated in the nuclei of human U2OS cells by UV radiation through the pores of polycarbonate filters. Endogenous p97 and a mildly overexpressed p97, tagged with a myc epitope (p97-myc), co-localized with CPDs ( Fig. 1a ), confirming that this segregase participates in the UV damage response. Time courses with endogenous p97 established the transient nature of this recruitment as all segregase complexes disappeared from the spots of UV damage formation within 24 h after irradiation ( Supplementary Fig. 1a, b ). Individual p97 subunits assemble to form hexamers that convert ATP hydrolysis into mechanical force by which target proteins are removed from cellular structures such as chromatin [25] , [26] . Therefore, the accumulation of p97 at CPD sites was markedly increased in the presence of an ATPase-inactive, dominant-negative mutant (p97 EQ) that still binds to ubiquitinated proteins but lacks segregase activity and, therefore, remains trapped on ubiquitinated substrates [37] ( Fig. 1a,b ). 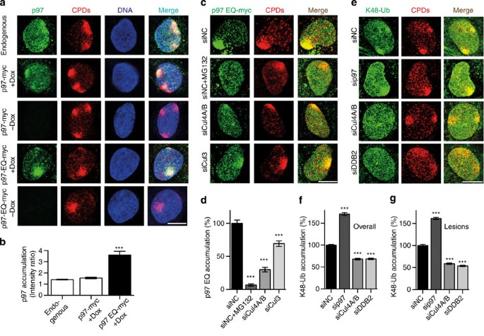Figure 1: Ubiquitin-dependent p97 recruitment to UV lesions. (a) Co-localization of p97 with CPDs in human cells. Mild expression of myc-tagged p97 (wild-type or p97 EQ) was induced with doxycycline (+Dox). Cells were probed 15 min after UV irradiation through micropore filters, whereby endogenous p97 was detected with anti-p97 antibodies and p97-myc with anti-myc antibodies. Scale bar, 10 μm. (b) UV-induced p97 re-localization shown as quantitative ratio of fluorescence at CPDs against surrounding nuclear areas (200 nuclei from two independent experiments); error bars, s.e.m., ***P<0.001 relative to wild-type (the unpaired two-tailedt-test was used for allP-value determinations). (c) Reduced recruitment of myc-p97 EQ to CPDs after treatment with MG132 or siRNA targeting the indicated cullins; siNC, non-coding control. (d) Quantification of p97 EQ at CPDs over three experiments (>300 nuclei), ***P<0.001 relative to siNC control (unpaired two-tailedt-test). (e) Increased K48-linked ubiquitin after treatment with siRNA targeting p97, CUL4A/B or DDB2. (f,g) Quantification (>300 nuclei from three experiments) of K48-linked ubiquitin in nuclei overall and at lesion sites, respectively. Figure 1: Ubiquitin-dependent p97 recruitment to UV lesions. ( a ) Co-localization of p97 with CPDs in human cells. Mild expression of myc-tagged p97 (wild-type or p97 EQ) was induced with doxycycline (+Dox). Cells were probed 15 min after UV irradiation through micropore filters, whereby endogenous p97 was detected with anti-p97 antibodies and p97-myc with anti-myc antibodies. Scale bar, 10 μm. ( b ) UV-induced p97 re-localization shown as quantitative ratio of fluorescence at CPDs against surrounding nuclear areas (200 nuclei from two independent experiments); error bars, s.e.m., *** P <0.001 relative to wild-type (the unpaired two-tailed t -test was used for all P -value determinations). ( c ) Reduced recruitment of myc-p97 EQ to CPDs after treatment with MG132 or siRNA targeting the indicated cullins; siNC, non-coding control. ( d ) Quantification of p97 EQ at CPDs over three experiments (>300 nuclei), *** P <0.001 relative to siNC control (unpaired two-tailed t -test). ( e ) Increased K48-linked ubiquitin after treatment with siRNA targeting p97, CUL4A/B or DDB2. ( f , g ) Quantification (>300 nuclei from three experiments) of K48-linked ubiquitin in nuclei overall and at lesion sites, respectively. Full size image Next to demonstrate that the p97 relocation to UV lesions is ubiquitin dependent, the nuclear compartment was depleted of its free ubiquitin pool by treatment with the proteasome inhibitor MG132 (ref. 38 ). The effective depletion of ubiquitin in the nuclear compartment is demonstrated, for example, by the missing ubiquitination of XPC following a standard UV insult ( Supplementary Fig. 1c ). This condition of nuclear ubiquitin depletion nearly abolished p97 EQ accumulation at CPD sites, confirming that protein ubiquitination is an essential signal for the p97 recruitment ( Fig. 1c,d ). Three different cullins (Cul3, Cul4A and Cul4B) are involved in K48-linked ubiquitination at UV damage [4] , [16] , [18] , [23] . Concomitant depletion of Cul4A and Cul4B by treatment with small interfering RNA (siRNA) caused a more severe reduction of p97 EQ relocation to CPDs than suppression of Cul3 ( Fig. 1c,d ; see Supplementary Fig. 1d for the efficiency of siRNA-mediated protein downregulation). A side-by-side comparison showed that Cul4A rather than Cul4B is primarily responsible for the p97 accumulation at CPDs ( Supplementary Fig. 1e,f ). That p97 has a role in the processing of ubiquitinated substrates at UV lesions was supported by comparing the amounts of nuclear K48-linked ubiquitin ( Fig. 1e ). Depletion of p97 by siRNA treatment increased the level of ubiquitin chains not only in the nucleus overall but also at CPD spots. Figure 1f,g shows the quantifications of K48-linked ubiquitin levels in the whole nucleus and at CPD spots, the latter determined by measuring the ratio of fluorescence signals relative to the nuclear surroundings. In conjunction, these findings indicate that p97 promotes the removal of Cul4A-ubiquitinated substrates from the chromatin overall but also from UV lesion sites. Recruitment of p97 segregase to UV lesions is DDB2 dependent A further siRNA screen (see Supplementary Fig. 2 for the efficiency of protein depletion) showed that the recruitment of p97 to UV lesions is primarily dependent on DDB2, the damage sensor subunit of the UV-DDB heterodimer ( Fig. 2a ). To a lesser degree, p97 is also recruited to UV damage by XPC, but no effect on the p97 localization was detected following depletion of XPA, which acts downstream of the early sensors DDB2 and XPC in the NER pathway ( Fig. 2a,b ). We therefore hypothesized that DDB2 is a main p97 substrate. 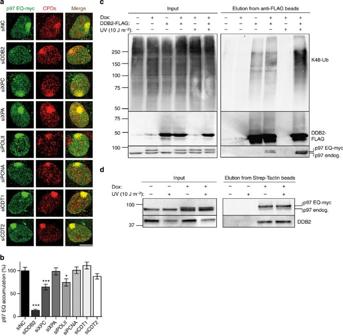Figure 2: Recruitment of p97 to UV lesions requires DDB2. (a) Co-localization of p97 EQ with CPDs in human cells treated with siRNA targeting the indicated proteins. Samples were probed 15 min after UV irradiation through micropore filters; scale bar, 10 μm. (b) Quantification of p97 EQ accumulation at CPDs as illustrated inFig. 2a. Error bars, s.e.m. (>300 nuclei from three experiments); *P<0.05, ***P<0.001 relative to siNC control (unpaired two-tailedt-test). (c) UV-stimulated interaction of p97 with a DDB2-containing complex. HEK293 cells were transfected to produce DDB2-FLAG and doxycycline-treated (Dox) for mild p97 EQ expression. DDB2-FLAG was pulled down from cell lysates using beads coated with anti-FLAG antibodies and eluates were analysed by immunoblotting against K48-ubiquitin, FLAG epitope and p97. Myc-tagged p97 migrates slower than the endogenous counterpart. (d) Interaction of DDB2 with the p97 complex. HEK293 cells were Dox for mild p97 EQ expression, and p97 EQ was pulled down from cell lysates using beads coated with Strep-Tactin. The resulting protein mixture was analysed by immunoblotting against p97 and DDB2. Figure 2: Recruitment of p97 to UV lesions requires DDB2. ( a ) Co-localization of p97 EQ with CPDs in human cells treated with siRNA targeting the indicated proteins. Samples were probed 15 min after UV irradiation through micropore filters; scale bar, 10 μm. ( b ) Quantification of p97 EQ accumulation at CPDs as illustrated in Fig. 2a . Error bars, s.e.m. (>300 nuclei from three experiments); * P <0.05, *** P <0.001 relative to siNC control (unpaired two-tailed t -test). ( c ) UV-stimulated interaction of p97 with a DDB2-containing complex. HEK293 cells were transfected to produce DDB2-FLAG and doxycycline-treated (Dox) for mild p97 EQ expression. DDB2-FLAG was pulled down from cell lysates using beads coated with anti-FLAG antibodies and eluates were analysed by immunoblotting against K48-ubiquitin, FLAG epitope and p97. Myc-tagged p97 migrates slower than the endogenous counterpart. ( d ) Interaction of DDB2 with the p97 complex. HEK293 cells were Dox for mild p97 EQ expression, and p97 EQ was pulled down from cell lysates using beads coated with Strep-Tactin. The resulting protein mixture was analysed by immunoblotting against p97 and DDB2. Full size image That p97 interacts with a DDB2-containing protein complex was shown by co-immunoprecipitation studies using human embryonic kidney 293 (HEK293) cells mildly expressing the p97 EQ mutant, tagged with a Strep peptide, together with FLAG epitope-tagged DDB2. A pull-down of DDB2-FLAG with anti-FLAG beads (coated with antibodies against the FLAG peptide) and analysis of the resulting eluates by western blotting demonstrated that p97 and DDB2 reside in the same multi-protein complex under unchallenged conditions ( Fig. 2c ). Such a constitutive association might reflect a basal turnover of DDB2 in human cells. In any case, the observed interaction between p97 and DDB2, the latter carrying K48-linked ubiquitin chains, was stimulated by UV radiation ( Fig. 2c ), supporting the notion that ubiquitinated DDB2 is a major p97 substrate upon UV exposure. This conclusion was supported by an inverse co-immunoprecipitation protocol, performed with the same HEK293 cells, whereby endogenous DDB2 was detected after pull-down of p97 EQ using Strep-Tactin beads that bind the Strep peptide of p97 ( Fig. 2d ). The strong dependence on DDB2 ( Fig. 2b ) and the differential role of E3 ligases in recruiting p97 ( Fig. 1d ) suggested a critical involvement of this segregase in global-genome NER activity regulated by UV-DDB and Cul4A. In comparison, only a minor proportion of p97 localizing to UV damage is apparently contributing to transcription-coupled NER. This view was confirmed by depleting POLII whose stalling at UV lesions triggers Cul3-mediated degradation [30] . In fact, suppression of POLII levels reduced the UV-dependent recruitment of p97 to the same small extent as the Cul3 depletion ( Fig. 2a,b ). Another scenario is that UV lesions block the DNA replication machinery [31] , [33] , [34] , [36] leading to degradation of the licensing factor CDT1 in a proliferating cell nuclear antigen (PCNA)- and CDT2-dependent manner [32] , [35] . However, depletion of none of these factors (PCNA, CDT1 or CDT2) reduced p97 recruitment to UV lesions ( Fig. 2a,b ), indicating that our assay, based on the induction of UV lesion spots, specifically monitors global-genome NER-related p97 functions. The p97 segregase extracts DDB2 and XPC from chromatin Next we tested how a depletion of p97 affects the homeostasis of DNA damage sensors in the NER pathway at the single-cell level. The siRNA-mediated downregulation of p97 resulted in increased recruitment (15 min after irradiation) and prolonged residence (180 min after irradiation) of DDB2 and XPC in UV-damaged areas ( Fig. 3a–c ), indicating that the p97 segregase extracts both sensors from chromatin. Retention of DDB2 in UV-irradiated chromatin was confirmed using cells expressing the p97 EQ mutant, which acts in a dominant-negative manner by generating inactive segregase complexes [37] ( Supplementary Fig. 3a,b ). That this segregase activity is dependent on prior substrate ubiquitination was additionally confirmed using a form of XPC that, as a result of its fusion with green fluorescent protein (GFP), is poorly ubiquitinated [17] , [39] . Unlike endogenous XPC ( Fig. 3c ), XPC-GFP was not removed from UV-damaged chromatin during the 180-min repair period ( Supplementary Fig. 3c,d ). The increased accumulation (after 15 min) and prolonged retention (after 180 min) under conditions of inactivated p97 is unique to DDB2 and XPC, as these effects do not extend to downstream NER factors such as XPB (a subunit of the TFIIH complex; Supplementary Fig. 3e,f ) or the ERCC1 subunit of the ERCC1-XPF endonuclease ( Supplementary Fig. 3g,h ). 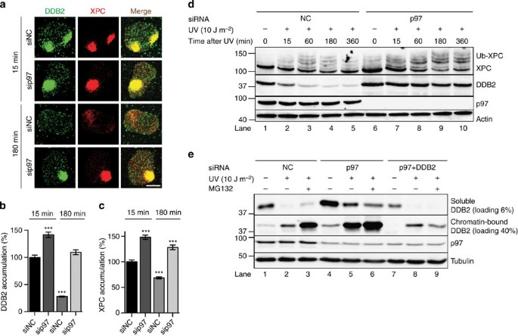Figure 3: The p97 segregase complex extracts DDB2 and XPC from chromatin. (a) Chromatin retention of DDB2 and XPC visualized 15 and 180 min after induction of UV damage spots in human cells treated with siRNA targeting p97 or non-coding (NC) control. Scale bar, 10 μm. (b,c) Quantification of DDB2 and XPC, respectively, in chromatin over three experiments (>300 nuclei). Error bars, s.e.m.; ***P<0.001 relative to siNC control (unpaired two-tailedt-test). (d) XPC hyperubiquitination and DDB2 degradation revealed by whole-cell immunoblot analysis after treatment with siRNA against p97 or NC control. (e) Levels of soluble (non-chromatin) and chromatin-bound DDB2 assessed in the respective cellular fractions. Figure 3: The p97 segregase complex extracts DDB2 and XPC from chromatin. ( a ) Chromatin retention of DDB2 and XPC visualized 15 and 180 min after induction of UV damage spots in human cells treated with siRNA targeting p97 or non-coding (NC) control. Scale bar, 10 μm. ( b , c ) Quantification of DDB2 and XPC, respectively, in chromatin over three experiments (>300 nuclei). Error bars, s.e.m. ; *** P <0.001 relative to siNC control (unpaired two-tailed t -test). ( d ) XPC hyperubiquitination and DDB2 degradation revealed by whole-cell immunoblot analysis after treatment with siRNA against p97 or NC control. ( e ) Levels of soluble (non-chromatin) and chromatin-bound DDB2 assessed in the respective cellular fractions. Full size image The homeostasis of XPC and DDB2 was further investigated using biochemical methods. Upon UV irradiation, XPC protein is partially and reversibly ubiquitinated, with a maximal extent of modification around 1 h after exposure [16] , [19] ( Fig. 3d , lane 3). Following p97 depletion, the proportion of ubiquitinated XPC was markedly increased and the ubiquitin modification remained for a longer time period of at least 6 h ( Fig. 3d , lanes 6–10). Conversely, DDB2 rapidly transfers to chromatin after UV radiation and is then degraded by proteasomal activity [24] ( Fig. 3d , lanes 1–5). This DDB2 clearance is inhibited by depletion of Cul4A ( Supplementary Fig. 4a ) or by depletion of p97 ( Fig. 3d , lanes 6–10). In chromatin, the inhibition of DDB2 breakdown by p97 depletion occurs to a similar extent as in the presence of the proteasomal inhibitor MG132 ( Fig. 3e , compare the chromatin-bound fractions of DDB2 in lanes 3 and 5). Accordingly, DDB2 persisted in the UV-damaged chromatin of p97-depleted cells ( Fig. 3e , compare the chromatin-bound fractions in lanes 2 and 5), whereas the combined depletion of p97 and DDB2 restored the lower level of DDB2 seen in control cells ( Fig. 3e , compare the chromatin-bound fractions of DDB2 in lanes 2 and 8). As the ubiquitination of DDB2 was not readily detected in cell lysates, to improve the visibility of this reaction, DDB2-FLAG was enriched by immunoprecipitation, under denaturing conditions, from transfected HEK293 cells using anti-FLAG beads. The resulting protein eluates were probed with antibodies against K48-linked ubiquitin, thus demonstrating that p97 depletion yields an increased level of ubiquitinated DDB2 relative to controls ( Supplementary Fig. 4b,c ). The stabilization of DDB2 against UV-induced degradation was confirmed using distinct siRNA sequences targeting p97 ( Supplementary Fig. 4d ) or by expressing the dominant-negative p97 EQ mutant ( Supplementary Fig. 4e ). In summary, these findings clearly show that p97 removes ubiquitinated DDB2 from UV lesions and thus facilitates its proteasomal breakdown. Adaptors for the recruitment of p97 to UV lesions Because the p97 segregase participates in multiple cellular processes, its substrate and site specificity is determined by adaptor proteins displaying both ubiquitin-binding and p97-interacting motifs [25] , [26] . Downregulation of the chromatin-related core adaptors Npl4 and Ufd1, by treatment with siRNA, completely abolished the recruitment of p97 to UV lesion spots ( Fig. 4a,b ). Instead, downregulation of UBXD1-mediating endolysosomal sorting did not interfere with this UV-dependent p97 recruitment. Similarly, downregulation of DVC1 (also known as Spartan or C1orf124) using the sequence siDVC_2, which resulted in efficient depletion ( Fig. 4c ), had no effect on the redistribution of p97 to UV lesion spots ( Fig. 4a,b ) despite the reported involvement of this adaptor in the DNA polymerase switch for translesion synthesis [31] , [33] , [34] , [36] . 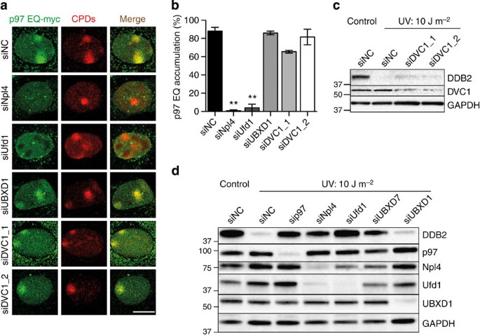Figure 4: Processing of DDB2 by the p97 segregase triggered by adaptors. (a) Co-localization of p97 EQ with CPDs in human cells treated with siRNA against the indicated adaptor proteins. The samples were probed 15 min after UV irradiation through micropore filters; scale bar, 10 μm. (b) Quantification of p97 EQ accumulation at CPDs as illustrated inFig. 4a. Error bars, s.e.m. (>300 nuclei from three experiments); **P<0.01, relative to siNC control (unpaired two-tailedt-test). (c) DDB2 degradation revealed by whole-cell immunoblot analysis after treatment with two different siRNA sequences against DVC1; siNC, non-coding control. GAPDH, glyceraldehyde 3-phosphate dehydrogenase as loading standard. (d) Inhibition of UV-triggered DDB2 degradation in cells treated with siRNA targeting p97 or the indicated adaptors. Figure 4: Processing of DDB2 by the p97 segregase triggered by adaptors. ( a ) Co-localization of p97 EQ with CPDs in human cells treated with siRNA against the indicated adaptor proteins. The samples were probed 15 min after UV irradiation through micropore filters; scale bar, 10 μm. ( b ) Quantification of p97 EQ accumulation at CPDs as illustrated in Fig. 4a . Error bars, s.e.m. (>300 nuclei from three experiments); ** P <0.01, relative to siNC control (unpaired two-tailed t -test). ( c ) DDB2 degradation revealed by whole-cell immunoblot analysis after treatment with two different siRNA sequences against DVC1; siNC, non-coding control. GAPDH, glyceraldehyde 3-phosphate dehydrogenase as loading standard. ( d ) Inhibition of UV-triggered DDB2 degradation in cells treated with siRNA targeting p97 or the indicated adaptors. Full size image Consistent with the different importance of these adaptors for the p97 recruitment during global-genome NER activity, we found that depletion of Npl4 or Ufd1, but not downregulation of UBXD1 or DVC1, stabilized DDB2 protein in UV-irradiated cells to a similar extent as observed in the absence of p97 ( Fig. 4c,d ). Also, in full accordance with its role in triggering DDB2 degradation, we found that Ufd1 interacts with a DDB2-containing protein complex in HEK293 cells ( Supplementary Fig. 4f ). These studies also identified the UBXD7 adaptor as an additional factor in the homeostasis of NER factors, as its downregulation results in partial protection of DDB2 from UV-induced breakdown ( Fig. 4d ). Taken together, our findings demonstrate that p97, upon recruitment by specific adaptors, namely the Ufd1-Npl4 heterodimer and UBXD7, processes K48-ubiquitinated DDB2 in UV-damaged chromatin. Excess of damage sensors reduces repair and genome stability In view of this crucial role of the p97 complex in the homeostasis of DNA damage sensors, we tested its contribution to global-genome NER activity. By monitoring the excision of UV lesions from chromosomal DNA, we observed that both the fast excision of 6-4PPs and the slow excision of CPDs [11] , [17] were attenuated by a p97 depletion in HeLa cells ( Fig. 5a,b ). Interestingly, the p97 downregulation caused inhibition of CPD excision in a similar manner as depletion of DDB2. That p97 functions as an accessory factor to facilitate NER activity explicitly in the physiologic chromatin context was supported by the finding that this segregase is not required for UV lesion excision from a transfected reporter plasmid ( Supplementary Fig. 5a ). This proficient repair of an ectopic and artificial substrate proofs that all NER factors are still present in p97-depleted cells, although they are unable to deploy their full activity on native chromosomes. Consistent with this compromised NER efficiency in the chromatin context, p97-depleted cells were hypersensitive to UV light ( Supplementary Fig. 5b ). 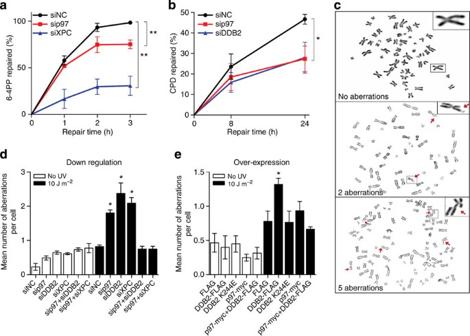Figure 5: An excess of damage sensors attenuates repair and causes genomic instability. (a) Excision of 6-4PPs in human cells treated with siRNA targeting p97 or XPC, used as comparator inflicting a severe repair defect; siNC, non-coding RNA control. Error bars, s.e.m. (n=3, each experiment with four replicates), **P<0.01 (unpaired two-tailedt-test). (b) Excision of CPDs upon treatment with siRNA targeting p97 or DDB2 (n=3, each experiment with four replicates), *P<0.05 (unpaired two-tailedt-test). In the case of CPDs, depletion of DDB2 is sufficient to compromise excision efficiency. (c) Metaphase spreads showing a progressively increasing genomic instability. Representative chromosomes are magnified in the inserts. (d) Chromosomal aberrations in cells treated with siRNA targeting the indicated proteins (n=3, 60 cells in a blinded analysis). *P<0.05 relative to siNC and cells with double depletion (unpaired two-tailedt-test). (e) Chromosomal aberrations in cells overexpressing the indicated proteins (n=3, 60 cells in a blinded analysis). *P<0.05 relative to cells expressing FLAG only and the double overexpressing cells (unpaired two-tailedt-test). Figure 5: An excess of damage sensors attenuates repair and causes genomic instability. ( a ) Excision of 6-4PPs in human cells treated with siRNA targeting p97 or XPC, used as comparator inflicting a severe repair defect; siNC, non-coding RNA control. Error bars, s.e.m. ( n =3, each experiment with four replicates), ** P <0.01 (unpaired two-tailed t -test). ( b ) Excision of CPDs upon treatment with siRNA targeting p97 or DDB2 ( n =3, each experiment with four replicates), * P <0.05 (unpaired two-tailed t -test). In the case of CPDs, depletion of DDB2 is sufficient to compromise excision efficiency. ( c ) Metaphase spreads showing a progressively increasing genomic instability. Representative chromosomes are magnified in the inserts. ( d ) Chromosomal aberrations in cells treated with siRNA targeting the indicated proteins ( n =3, 60 cells in a blinded analysis). * P <0.05 relative to siNC and cells with double depletion (unpaired two-tailed t -test). ( e ) Chromosomal aberrations in cells overexpressing the indicated proteins ( n =3, 60 cells in a blinded analysis). * P <0.05 relative to cells expressing FLAG only and the double overexpressing cells (unpaired two-tailed t -test). Full size image Given that the p97 segregase (i) processes K48-ubiquitinated DDB2 and XPC proteins; (ii) positively regulates NER activity in chromatin; and (iii) promotes cell survival after UV exposure, we finally tested whether this newly discovered regulation of DDB2 and XPC homeostasis contributes to genome stability by monitoring aberrations in metaphase chromosomes ( Fig. 5c ). We used HEK293 cells, unable to respond to UV damage with p53- and p21-dependent checkpoints [40] , to exclude possible indirect and confounding effects from DNA damage-induced cell cycle arrest. An increased frequency of chromosomal aberrations occurred in p97-, DDB2- and XPC-depleted cells both under unchallenged conditions and, to a more pronounced degree, upon UV radiation ( Fig. 5d ; see Supplementary Fig. 5c for the corresponding protein levels). Importantly, the genome instability following p97 depletion in UV-irradiated cells, but not in unchallenged cells, was reversed by concurrent downregulations, by siRNA, that reduce the level of DDB2 or XPC ( Fig. 5d ). These results suggested that a tight control of damage sensor levels in chromatin is essential for genome stability after UV radiation. As the siRNA-mediated depletion of DDB2 and XPC is not complete (see for example the remaining chromatin-bound fraction of DDB2 in Fig. 3e , lane 8), the reduced levels of these sensors are still adequate in a p97-deficient background to mediate a suitable NER response that prevents the formation of chromosomal aberrations upon infliction of UV damage. The previous results indicate that an uncontrolled accumulation of DDB2 or XPC in chromatin is detrimental. If this hypothesis were correct, then excessive expression of such a damage sensor would be sufficient to cause genome instability in a background of normal p97 activity. This challenging concept was confirmed by demonstrating that overexpression of wild-type DDB2 but not overexpression of the DNA damage recognition-defective K244E mutant [41] , both as FLAG-tagged constructs, inhibited the excision of 6-4PPs and CPDs ( Supplementary Fig. 5d,e ) and enhanced the frequency of chromosomal defects upon UV irradiation relative to control cells containing only the FLAG tag ( Fig. 5e ). Subsequently, double transfection experiments were carried out to induce the combined overexpression of both DDB2-FLAG and p97. The outcome of these double transfections ( Fig. 5e ) demonstrates that, by extracting the surplus of DDB2 from chromatin (see Supplementary Fig. 5f for DDB2-FLAG levels in and out of chromatin), a concomitant overexpression of the p97 segregase is able to reverse the chromosomal instability triggered by DDB2-FLAG present in excess. The enhancement of p97 amounts reached in these transfection-mediated overexpression experiments is illustrated in Supplementary Fig. 5g . To conclude, these findings show that increased levels of chromatin-bound DDB2 compromise genome stability only when they exceed the rate-limiting turnover capacity of the p97 segregase complex. This report identifies the p97 segregase machinery as a critical factor in the global-genome NER response that constitutes the main DNA repair system for protection from sunlight-induced skin mutagenesis and cancer. We show that the functional consequences of a downregulated p97 protein expression in human cells include UV hypersensitivity, a reduced rate of photoproduct excision and, consequently, an increased frequency of UV-induced chromosomal aberrations. The earliest DNA damage sensors in the global-genome NER pathway, DDB2, becomes a substrate of the p97 segregase when it is modified by Cul4A ligase-mediated ubiquitination in response to UV light. Depletion of XPC reduced the p97 accumulation at UV lesion sites, indicating that this simultaneously ubiquitinated partner is also a direct substrate of the p97 segregase. Thus, our findings imply that a key function of the ubiquitin modification is to prime these initial DNA damage sensors and NER initiators for subsequent extraction from chromatin. Along with UV-DDB and Cul4A ubiquitin ligase activity, recruitment of the p97 segregase to UV photoproducts depends on the ubiquitin-binding adaptors Npl4, Ufd1 and UBXD7, which are mediators of chromatin-associated p97 functions and, hence, confer substrate and site specificity to the p97 machine [25] , [26] . Even though DDB2 is needed for the efficient detection and excision of UV lesions, particularly of CPDs, ubiquitination leads to its degradation often within a few hours after exposure to UV light [24] , [42] , [43] , but the actual trigger and scope of this apparently paradoxical breakdown of a lesion recognition subunit was unclear. Similarly, how the reversible ubiquitination of XPC protein influences the NER mechanism was poorly understood, although a widely accepted hypothesis is that this transient modification increases the binding affinity of XPC for DNA [16] . The newly identified role of p97 in the processing of ubiquitinated DDB2 and XPC provided a fresh strategy to investigate the impact of ubiquitin-mediated DDB2 degradation as well as the role of XPC ubiquitination. Our study is the first to show that, in the context of chromatin, a strict spatiotemporal control of the DNA lesion-associated homeostasis of DDB2 and XPC by the p97 segregase is critical for efficient NER activity ( Supplementary Fig. 6 ). This conclusion is supported by the finding that overexpression of DDB2, resulting in prolonged binding of this damage sensor to lesion sites, inhibits the NER process rather than leading to a repair stimulation. Interestingly, the deleterious cellular end point (chromosomal aberrations) resulting from a deficient p97 function could be avoided by partial downregulation of DDB2 and XPC protein levels, confirming that an excess of these factors in the damaged chromatin of cells recovering from UV radiation is detrimental to genome stability. This is further demonstrated by the fact that overexpression of DDB2 is sufficient to boost up genome instability in UV-irradiated cells, and that this harmful outcome can be prevented by stimulating its degradation through concomitant p97 overexpression. In summary, the paradigm of DDB2 homeostasis illustrates how both low and high levels of DNA damage sensors cause slow repair and genome instability ( Supplementary Fig. 6 ). DDB2 stimulates the excision of UV lesions [11] , [12] , [13] , [14] but, if bound to damaged chromatin in excess because of a failure in its extraction and degradation, this same sensor acquires genotoxic properties culminating in chromosomal aberrations. Regulatory roles of DDB2 beyond its NER function have been identified in the processes of apoptosis [44] , [45] , cellular senescence [46] , epithelial-to-mesenchymal transitions [47] , breast tumour invasion [48] and alkylating drug resistance [49] . Therefore, the p97-directed control of DDB2 levels in damaged chromatin is of general importance for the understanding of genome dynamics, tumour development and cancer treatment [50] . Cell lines Parental U2OS, HEK293 and HeLa cells, obtained from American Type Culture Collection, were grown in the dark using Dulbecco’s modified Eagle medium supplemented with 10% fetal calf serum (FCS; Gibco), 100 U ml −1 penicillin and 100 μg ml −1 streptomycin. In addition, 100 μg ml −1 hygromycin B and 100 μg ml −1 Zeocin were used in the case of stably transfected p97-myc U2OS cells, whereas 100 μg ml −1 hygromycin B and 15 μg ml −1 blasticidin S were used for stably transfected p97-myc-Strep HEK293 cells. U2OS cell lines, stably transfected with the inducible complementary DNA for wild-type p97 and p97 EQ, both displaying the myc epitope, were provided by Weihl and coworkers [51] . The corresponding HEK293 cells were designed as described in the Flip-In T-Rex 293 system protocol (R780-07; Invitrogen) [27] . Mild expression was achieved by induction with 1 μg ml −1 doxycycline for 24 h (wild-type p97) and 18 h (p97 EQ). All cell lines were tested negative for mycoplasma contamination. siRNA transfections The siRNA sequences were purchased from Qiagen, Microsynth or Invitrogen ( Supplementary Table 1 ). Transfections were performed with Lipofectamine RNAiMAX according to the manufacturer’s protocol (Invitrogen). The siRNA concentrations were 16 nM for the silencing of p97, 20 nM for adaptors and 10 nM for all other targets (siRNA sequences are listed in Supplementary Methods ). Cells were analysed 72 h after siRNA transfections. Plasmids and cloning The BamHI restriction was used to obtain the human DDB2 complementary sequence from plasmid DDB2-GFP-C1 (a gift from Dr S. Linn, University of California, Berkeley, CA, USA) for insertion into the expression vector p3XFLAG-CMV-14 (Sigma). The K244E mutant [41] was generated by site-directed mutagenesis using the QuickChange site-directed mutagenesis kit (Stratagene). The plasmid pcDNA5frt/to-p97wt for expression of wild-type p97 was described earlier [27] . A derivative resistant to siRNA against p97 was generated on the basis of the above-mentioned construct using QuickChange with the following primers: forward, 5′-AGCCGATTCAAAAGGTGATGATTTATCCACGGCTATCCTAAAGCAAAAGAACCG TCCCAATCGG-3′; reverse: 5′-CCGATTGGGACGGTTCTTTTGCTTTAGGATAGCCGT GGATAAATCATCACCTTTTGAATCGGCT-3′. Plasmid pEGFP-C1-Ufd1, used for ectopic expression of the Ufd1 adaptor, was a gift from Dr H. Meyer, University of Duisburg-Essen, Germany. Plasmid transfections DNA transfections were performed with FuGENE HD reagent according to the manufacturer’s protocol (Roche). Cells were transfected at 20% confluency and analysed 72 h later, unless otherwise indicated in figure legends. UV irradiation Exposure of the cells to UV-C light was carried out with a germicidal lamp (wavelength 254 nm) after washing with phosphate-buffered saline (PBS). Local damage was generated by irradiation with 100 J m −2 through a 5-μm polycarbonate filter (Millipore) [52] . Cells were recovered for the indicated time periods under normal culture conditions before they were processed for further analyses. Protein synthesis was inhibited by addition of cycloheximide (100 μg ml −1 , Sigma) for 30 min before UV irradiation. Immunofluorescence microscopy studies Cells were grown on glass coverslips to 80% confluency. Pre-extraction buffer (25 mM HEPES, pH 7.5, 50 mM NaCl, 1 mM EDTA, 3 mM MgCl 2 , 300 mM sucrose and 0.5% (v/v) Triton X-100) was added for 2.5 min at 4 °C. Thereafter, cells were fixed with 4% paraformaldehyde (w/v) for 15 min and permeabilized for 20 min with PBS containing 0.1% (v/v) Tween 20. Primary antibodies (listed in Supplementary Table 2 ) were diluted in PBS with 5% FCS and applied for 1 h at 37 °C after a 30-min blocking step with PBS containing 20% FCS. Secondary antibodies, diluted in PBS with 5% FCS, were added for 30 min at 37 °C after washing with PBS-Tween 20 and blocking for 20 min with PBS containing 20% FCS. DNA was stained with 4′,6-diamidino-2-phenylindole (DAPI; 0.2 μg ml −1 ) for 10 min. Images of immunostained cells were taken with an SP5 confocal microscope (Leica) and analysed with the ImageJ software. The accumulation of proteins at UV lesion sites was expressed as the ratio of fluorescence signal intensity at the damage site to the respective intensity in the remaining nuclear area after subtraction of the background intensity detected outside of the nucleus. Only in Fig. 1b , protein accumulation is presented directly as intensity ratios, whereas in all subsequent figures the results are expressed as the percentage of the ratio obtained with the indicated control treatment. Immunoblotting Cells were treated as indicated, washed with Puck’s-EDTA and lysed in 100 μl of 1% Triton buffer (150 mM KCl, 25 mM Tris–HCl, pH 7.5, 5 mM MgCl 2 , 2 mM β-mercaptoethanol, 5% glycerol, 1 mM N -ethylmaleimide, 1% (v/v) Triton X-100 and protease inhibitor cocktail (Roche)). Protein concentrations were measured by Bradford analysis [53] , Laemmli sample buffer [54] was added and boiled for 10 min at 95 °C. In each case, 50 μg of sample proteins were separated on 4–20% Criterion TGX stain-free precast gels (Bio-Rad) and transferred to polyvinyldene fluoride membranes using a Turbo transfer device (Bio-Rad). Antibodies used for immunoblotting are listed in Supplementary Table 2 , and all full blots are shown in Supplementary Figs 7 and 8 . Chromatin digestion Chromatin was dissected as described previously [17] . Briefly, cells were grown to confluency on 8.5 cm dishes, UV-irradiated with the indicated UV doses and lysed on ice with NP-40 buffer (25 mM Tris–HCl, pH 8.0, 0.3 mM NaCl, 1 mM EDTA, 10% (v/v) glycerol, 1% (v/v) NP-40, 0.25 mM phenylmethylsulfonyl fluoride and EDTA-free protease inhibitor cocktail (Roche)). Cell lysis was carried out for 30 min on a turning wheel. Free, non-chromatin-bound proteins were recovered by centrifugation (10 min, 15,000 g ). Micrococcal nuclease (MNase; New England Biolabs) digestion was then accomplished for 20 min at 37 °C. For that purpose, the chromatin-containing pellet was suspended in CS buffer ((20 mM Tris–HCl, pH 7.5, 100 mM KCl, 2 mM MgCl 2 , 1 mM CaCl 2 , 0.3 M sucrose and 0.1% (v/v) Triton X-100)) ref. 55 and supplemented with × 10 reaction buffer (500 mM Tris–HCl, pH 7.9, 50 mM CaCl 2 ), bovine serum albumin (1 mg ml −1 ) and MNase (4 U μl −1 ). Solubilized proteins were recovered by centrifugation (10 min, 15,000 g ) after adding EDTA (5 mM) to stop the nuclease digestion. Affinity purification of DDB2-FLAG complexes Stable, inducible p97 EQ-Strep HEK293 cells were transfected with the vector for expression of DDB2-FLAG. The expression of p97 was induced by the addition of doxycycline as indicated in the figure legends. Cell fractions after MNase digestion were pooled (free non-chromatin-bound fraction containing soluble proteins and MNase-solubilized proteins), and the resulting mixture was incubated with anti-FLAG M2 affinity gel (Sigma) in the presence of immunoprecipitation buffer (150 mM NaCl, 50 mM Tris–HCl, pH 7.5, 5 mM MgCl 2 , 1% (v/v) NP-40, 2 mM β-mercaptoethanol, 5% (v/v) glycerol, EDTA-free protease inhibitor cocktail (Roche) and 10 mM N -ethyl maleimide). The gel beads were washed with TNET buffer (50 mM Tris–HCl, pH 7.4, 150 mM NaCl, 5 mM EDTA, 0.5% (v/v) Triton X-100), TNE buffer (50 mM Tris–HCl, pH 7.4, 100 mM NaCl, 0.1 mM EDTA) and H 2 O after an overnight incubation. The subsequent elution was performed with 0.3 μg μl −1 3XFLAG peptide (Sigma) for 1 h at 4 °C on a shaker plate. For the extraction of ubiquitinated DDB2-FLAG in denaturing conditions, cells were lysed (50 mM Tris–HCl, pH 6.8, 5 mM DTT and 1% (w/v) SDS) and sonicated before the solution was diluted four times with NP-40 buffer (25 mM Tris–HCl, pH 8.0, 0.3 mM NaCl, 1 mM EDTA, 10% (v/v) glycerol, 1% (v/v) NP-40, 0.25 mM phenylmethylsulfonyl fluoride and EDTA-free protease inhibitor cocktail (Roche)) and subjected to immunoaffinity purification with anti-FLAG M2 affinity gel as described above. Affinity purification of p97 EQ-Strep complexes Inducible p97 EQ-Strep from HEK293 cells was purified by Strep-Tactin sepharose beads (IBA Technologies) according to the manufacturer’s protocol, in the presence of buffer containing 120 mM NaCl, 50 mM Tris–HCl, pH 7.5, 5 mM MgCl 2 , 0.25% (v/v) NP-40, 2 mM mercaptoethanol, 5% (v/v) glycerol and protease/phosphatase inhibitor (Roche). After this pull-down, beads were washed, samples were boiled in loading buffer and the proteins were analysed by polyacrylamide gel electrophoresis and immunoblotting. Quantification of UV lesions To monitor the excision of UV lesions, antibodies against 6-4PPs and CPDs (Cosmo Bio) were used in a quantitative enzyme-linked immunosorbent assay [17] according to the manufacturer’s instructions. Briefly, DNA purified from the whole genome (DNeasy Blood and tissue kit, Qiagen) was denatured by heating (99 °C, 10 min) followed by a 15-min incubation on ice. A volume of 50 μl per well of denatured DNA (4 μg ml −1 for 6-4PP detection, 200 ng ml −1 for CPD detection) was distributed into a 96-well microtiter plate (Greiner) coated with protamine sulphate (Sigma) and dried overnight at 37 °C. The DNA-coated plates were washed five times with PBST (0.05% (v/v) Tween 20 in PBS) and blocked with 2% FCS in PBS at 37 °C for 60 min. The antibodies against either 6-4PPs (64M-2) or CPDs (TDM-2) were used for 30 min (37 °C) at dilutions of 1:2,000 and 1:5,000, respectively. Primary antibodies bound to DNA molecules were recognized by biotin-labeled F(ab’) 2 fragments of anti-mouse IgG (1:2,000; B-11027; Invitrogen) added for 30 min at 37 °C. After washing the plates, 100 μl of a peroxidase–streptavidin conjugate (1:10,000; Invitrogen) was distributed into each well. The reaction was started by adding 0.5 mg ml −1 o -phenylenediamine, 0.007% H 2 O 2 and citrate-phosphate buffer (50 mM Na 2 HPO 4 , 24 mM citric acid, pH 5.0), stopped with 50 μl of 2 M H 2 SO 4 , and monitored by measuring the absorbance at 492 nm in a PLUS384 microplate spectrophotometer (Molecular Devices). Chromosome analysis HEK293 cells lacking p53- and p21-dependent checkpoint activation [40] were treated with siRNA for 72 h or, alternatively, transfected with overexpression plasmids. Cells were subsequently UV irradiated with 10 J m −2 , or left untreated, exposed to 100 nM nocodazole for 4 h, lysed with hypotonic solution (0.4% KCl) for 15 min and fixed in methanol:acetic acid (3:1). Cell suspensions were spread on a slide, air-dried and stained in Giemsa solution for 2 min. Metaphase spreads were detected using an Axio imaging 2 microscope (Zeiss, Jena, Germany) and captured using the Ikaros software (Metasystems, Altlusheim, Germany). Host-cell reactivation assay HeLa cells were grown to 10–20% confluency in a six-well dish and transfected with siRNA targeting the indicated proteins. Following 72 h, DNA transfections were carried out with 0.9 μg UV-irradiated pGL3 (254 nm wavelength, 1,000 J m −2 ) and 0.1 μg non-irradiated pRL-TK (FUGENE HD, Roche). Cells were lysed after another 18 h incubation period according to the manufacturer’s protocol (Dual Luciferase Assay, Promega). Ratios between Photinus and Renilla luciferase activity were determined in triplicates with a microtiter plate luminometer (Dynex). Survival (colony-forming) assay HeLa cells were transfected with siRNAs as previously described, UV-treated at increasing doses, seeded in different dilutions and incubated in cell culture medium for 7 days at 37 °C to allow for colony formation. Colonies were stained with 0.5% (w/v) crystal violet in 80% ethanol and counted. Statistics Mean values and s.e.m. are shown for each experiment. Differences between groups were calculated in GraphPad Prism 6 using unpaired, two-tailed, t -tests. P values expressed as * P <0.05, ** P <0.01 and *** P <0.001 were considered to be significant. Between-group variances were similar and data were symmetrically distributed. In immunofluorescence studies, three independent experiments were performed and at least 100 random samples per experiment were scored in each group. To illustrate the sample size calculations for adequate statistical power, significance levels were set to 0.05, power levels to 0.9 and effect size to 0.5 according to the estimated mean values and s.d. The R statistical software version 3.0.1 was used to calculate sample size using two-sample t -test for power analysis (pwr package) yielding a sample size of 86. Analogous power calculations were carried out for all other assays. In the enzyme-linked immunosorbent assay measurements, three independent experiments with four technical replicates were performed for each treatment. In chromosome analyses, 60 metaphase spreads were scored for chromosomal aberrations in three independent, blindly performed experiments. In colony-forming assays, three independent experiments with three technical replicates were performed for each treatment. How to cite this article: Puumalainen, M.-R. et al . Chromatin retention of DNA damage sensors DDB2 and XPC through loss of p97 segregase causes genotoxicity. Nat. Commun. 5:3695 doi: 10.1038/ncomms4695 (2014).